Community voices: the importance of diverse networks in academic mentoring Multiple efforts have been made by institutions, societies, and organizations to offset gender disparity and exclusion of underrepresented minority scientists (URMs, i.e. racial/ethnic and gender groups constituting a lower proportion in the field than in the general population). Programs addressing gender bias and lack of diversity are slowly, but increasingly, addressing ingrained sexism and ableism in STEM fields and academia [1] , [2] , [3] . However, institutions and funding agencies should continue to invest in minimizing gender-specific obstacles; for example, promoting work-life balance; equalizing salaries, promotions, and start-up packages. Institutions must also address cultural taxation, discrimination, and isolation of URMs [4] , [5] , [6] . Further, institutions should act as tools of social justice by acknowledging women and URMs in leadership positions where they were historically ignored; honoring them with awards and nominations; and promoting and compensating them when serving as role models and mentors. Here, we recommend tangible action focused on the latter. Mentor relationships are crucial to retention, success, and wellbeing of women and URMs in academia. Mentoring not only provides professional support, guidance, information, and advice; mentoring also offers templates of the behaviors that are needed to achieve success in the field [7] , [8] . Effective mentorship requires a unique personal relationship between individuals at different career stages, with the potential of benefiting the career advancement of both the mentor and the mentee [9] . Further, mentorship is distinct from supervision: “Mentoring is an opportunity to connect meaningfully with individuals in service to their pursuit of personally-defined goals or aspirations” [10] . Thus, mentorship is not automatically achieved in a supervisor-supervisee relationship [11] . However, even when dyadic mentor-mentee relationships have been shown highly beneficial [12] , the traditional model of mentoring can be insufficient to ensure retention, success, and wellbeing of underrepresented groups (by either race/ethnicity or gender identity in academia) [13] , [14] , [15] . Women and URMs face many obstacles during their academic careers, in great part due to ingrained institutional disparity: decreased recognition in publications, fewer citations of papers authored by them, lower research funding allocations, and greater academic and domestic responsibilities [4] , [16] , [17] , [18] , [19] , [20] . These biases lead to gender and ethnic underrepresentation in academia, particularly at senior levels [21] , [22] . Indeed, women and URMs are less represented at later stages in the career path (a phenomenon known as ‘the leaky pipeline’ [23] ). A network of diverse mentors may support achieving long-term career goals, advancement, and retention of both mentors and mentees, thus synergistically enhancing diversity, equity, and inclusion (DEI) initiatives and perpetuating a virtuous cycle of enriched mentoring [8] . Programs focusing on building diverse mentorship networks have been effective in promoting the success of women and other URMs in Science, Technology, Engineering and Mathematics (STEM) fields [24] , [25] , [26] , [27] . Cross-cultural mentoring relationships have been particularly successful when they included strategies to foster mentors’ awareness, sensitivity, and commitment to their mentees [15] . In this context, improved culturally and socially diverse mentorship can enable institutions to effectively increase DEI and overcome bias in STEM fields and academia. While multiple organizational efforts are focused on increasing DEI, the actual practice of these efforts is challenging. To achieve the goal of increased DEI, we suggest that institutions aim to: (1) emphasize mentoring strategies to increase DEI, especially those that address gender bias and URM exclusion, (2) promote multi-mentor programs and acknowledge their utility in increasing DEI, and (3) reference examples of diverse, institutional mentoring efforts. Having diverse role models and mentors can be transformative and enhance academic performance, especially for women and URM mentees. Retention, motivation, and persistence in STEM fields and academia can be positively influenced by mentorship [25] . This is particularly impactful when female students and URMs are introduced, at an early undergraduate stage, to role models and mentors by whom they feel represented [26] , [28] . For instance, different mentorship programs focused on equity and inclusion of URMs have proven to be effective long after the relationship ended, sustaining the retention and success of underrepresented scientists [5] , [25] , [28] , [29] , [30] . For mentorship to be impactful for academic advancement though, the individuals in the relationships cannot be separated from their cultural and societal backgrounds. Mentors and mentees pairing often reflect unconscious biases [31] (e.g., majority-culture mentors interacting with mentees with ethnic, religious or gender affinities in ways that reflect majority-culture priorities rather than tailoring mentoring to these URM mentees’ priorities). Thus, active efforts from institutions are required to counteract the systemic inequities. Such efforts, particularly when formalized as programs, expand opportunities for both mentors and mentees to be more productive and innovative [8] , [31] . For example, women usually devote a substantial part of their time, more than men, to mentorship and teaching [27] . This imbalance can reduce publication and grant success which then contributes to unequal attrition of women mentors. Further, if women and URMs are less represented in advanced career stages, diverse mentors and whole lines of research are less present in STEM, which increases the burden on the available mentors even more. A pyramidal structure toward less representation of women and URMs in senior positions thereby undermines efforts to overcome mentorship and research biases while exacerbating the burden on those few women and URMs who are retained long enough to become mentors [9] , [13] , [14] , [19] , [22] , [23] , [27] , [29] . One solution is promoting mentorship networks, involving multiple mentor-mentee relationships, to increase collective performance by magnifying resources [8] , [24] , [32] , [33] . In effective mentorship networks, mentorship extends beyond the relationships of mentors and their direct mentees. Indeed, mentors can be purposely picked outside the mentee’s direct advisory network [11] . 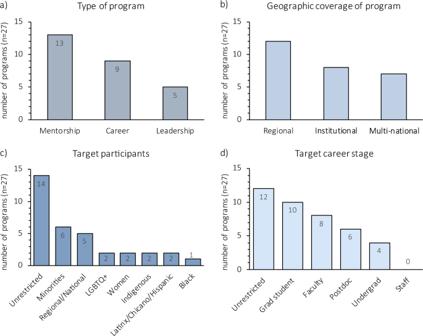Fig. 1: Attributes of career development, leadership and mentorship programs from around the world. Graphs represent the number of identified programs according toatype of program,bgeographic coverage of the program,ctarget participants, anddtarget career stage. Most programs we reviewed focus on mentorship, are offered regionally, are not limited to specific target groups, and emphasize faculty and postdoc career stages. Notably, no programs specifically target staff (non-faculty, university employees), despite evidence that staff and contingent faculty roles (e.g., adjuncts, non-tenure-track) do extensive service in mentoring and provision of DEI services in academia. Also, most programs include multiple target categories, so totals are >n in figure sectionscandd. 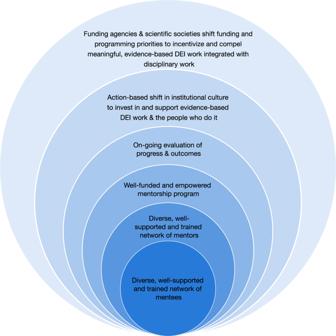Fig. 2: Framework to build diverse multi-mentors networks. Establishing effective programs that promote diverse multi-mentor networks -- in which mentees and mentors are supported and trained to (1) build healthy relationships, (2) develop professionally, and (3) achieve success – is a layered process that depends on many embedded factors:aDEI assessment implemented by institutions, funding agencies, scientific societies, and the community;bpolicy and work culture changes to promote evidence-based DEI work;ccontinuous support and evaluation of program implementation, progress, and outcomes; anddreassessment, adaptation, and reevaluation of programs to empower mentorship networks. As a dynamic system, all components feed from and are informed by the others. Building a multi-mentor network is an emergent property of other available systems, as programs often center around matching mentor/mentee pairs (Table 1 ). Such programs frequently offer the possibility of establishing peer and group mentoring relationships (for example, National Research Mentoring Network [34] ), thereby building networks for people in both shared and different career stages. However, we note a gap in formal programs: resources and recognition are needed for establishing these multi-mentor networks (Table 1 and Fig. 1 ). First, effective mentorship programs require changing institution-wide practices and interactions to challenge systemic inequalities on all organizational levels [35] . For example, institutional policies can mitigate the overburden of mentoring by women and URMs (which, as noted, exacerbates attrition) by establishing review and promotion guidelines and responsibility re-allocation to encourage and credit mentors who participate in diverse mentoring programs [36] , [37] , [38] . While some solutions can be generalized, each institution faces unique circumstances that require specific actions. Although doing so is challenging, not addressing these issues in local contexts may cause even the best program to fail. Table 1 Career development, leadership and mentorship programs: examples from around the world. Full size table Fig. 1: Attributes of career development, leadership and mentorship programs from around the world. Graphs represent the number of identified programs according to a type of program, b geographic coverage of the program, c target participants, and d target career stage. Most programs we reviewed focus on mentorship, are offered regionally, are not limited to specific target groups, and emphasize faculty and postdoc career stages. Notably, no programs specifically target staff (non-faculty, university employees), despite evidence that staff and contingent faculty roles (e.g., adjuncts, non-tenure-track) do extensive service in mentoring and provision of DEI services in academia. Also, most programs include multiple target categories, so totals are >n in figure sections c and d . Full size image Furthermore, once efforts and programs are established, their methods and outcomes must be continuously monitored and evaluated to ensure institutions reassess successful or failed activities dynamically and responsively. Effectiveness may also be achieved when pre-established programs are synchronized and interconnected, thereby helping to identify diverse mentors for specific aspects of academic life. Successful programs will offer continuous support throughout the academic path, enabling professional development of both mentors and mentees and empowering diverse groups by promoting access to available resources and providing appropriate recognition. Building a diverse and inclusive network helps promote a sense of identity and community that counteracts feelings of isolation often experienced by scientists throughout their careers [39] . Mentoring networks, including peer mentors, should also be encouraged because they are more balanced in power and transparency, and less hierarchical [40] , [41] . Peer mentor networks can be particularly effective for tackling same-career-stage challenges and opportunities [28] , [33] , [42] . All these efforts should be accompanied by human resources training and implementing codes of conduct detailing best practices to make the whole experience for mentors and mentees more enjoyable and successful [36] , [43] , [44] . By diversifying the academic community with which mentors and mentees actively engage, scientific advancement can be achieved in a nurturing environment that can have a strong, positive impact on productivity [25] , [32] , [33] . Therefore, fostering mentorship networks should be a high priority for any academic institution undertaking DEI efforts. Though not widely adopted, there are models for this approach worldwide (Table 1 ). Select academic institutions, professional societies, and conference organizers offer training programs to promote successful mentorship relationships that subsequently support diverse and more inclusive work environments. Although the outcomes of many programs have not yet been quantified or evaluated, some programs have minimized gender-specific barriers and reduced exclusion of URMs [24] , [45] , [46] , [47] . Evaluating outcomes of mentorship programs remains challenging; traditional quantitative approaches may not be sufficient to capture how programs promote careers in nuanced, individualized ways that transcend the normative metrics of academic productivity and research impact (which themselves can promote inequalities) [48] . Even though assessment for such programs is challenging, the outcomes can be qualified within a range of acceptable parameters assessing individual, group, and institutional growth [24] , [45] , [46] , [47] . Since women and URM scientists are generally more involved in formal and informal mentoring activities [27] , overburdening may be detrimental for program implementation and success. Therefore, evaluations should be accompanied by incentive programs for mentors, such as release from administrative and departmental duties and provision of funding awards. Funding agencies should also: (1) explicitly include DEI requirements in their guidelines for grant spending, (2) provide resources to support reviewers, grantees, and institutions in the implementation of mentoring networks that could arise within institutions or from collaboration networks, and (3) hold grantees accountable if not following those guidelines. Policy changes and active implementation of programs that promote effectively, diverse mentorship networks can help women and URMs to fully achieve their potential as scientists. And yet, we see a disheartening lack of resources directed to career development, leadership, and mentorship programs in some regions (Fig. 1 ). For example, our own experiences and observations indicate there is a particular dearth of these resources across the Global South (i.e. Latin America, Africa, and South Asia; Fig. 1 ). Indeed, other than collaboration groups or a few institutional efforts, many academics worldwide have no support to successfully navigate the mentoring process, establish healthy relationships with their mentors or mentees, or even have a resource to which they can turn should problematic situations arise. A diverse environment improves working and learning experiences for the people involved, brings new perspectives to research, encourages more people to work in STEM fields and academia, and improves opportunities for everyone involved. To achieve this goal, we urge all agencies, foundations, institutions, and societies to use the many existing examples to inform their development of programs to generate effective mentoring relationships within their sphere of influence. We also present a step-by-step framework to diversify and build mentorship networks that includes all the aspects discussed in this commentary (Fig. 2 ). Building effective, diverse, multi-mentor networks can only work when programs are informed and accompanied by institution-wide DEI policy implementation, reflect diversity of the community in which institutions are embedded, and synchronize support for all organizational and career levels. Healthier work environments, more inclusive science training, and better outcomes for professionals from all backgrounds would ideally ensue as successful program implementation broadens, creating a virtuous cycle of enriched mentoring for future generations. Fig. 2: Framework to build diverse multi-mentors networks. Establishing effective programs that promote diverse multi-mentor networks -- in which mentees and mentors are supported and trained to (1) build healthy relationships, (2) develop professionally, and (3) achieve success – is a layered process that depends on many embedded factors: a DEI assessment implemented by institutions, funding agencies, scientific societies, and the community; b policy and work culture changes to promote evidence-based DEI work; c continuous support and evaluation of program implementation, progress, and outcomes; and d reassessment, adaptation, and reevaluation of programs to empower mentorship networks. As a dynamic system, all components feed from and are informed by the others. Full size image